Ordered bilayer ruthenium–platinum core-shell nanoparticles as carbon monoxide-tolerant fuel cell catalysts Fabricating subnanometre-thick core-shell nanocatalysts is effective for obtaining high surface area of an active metal with tunable properties. The key to fully realize the potential of this approach is a reliable synthesis method to produce atomically ordered core-shell nanoparticles. Here we report new insights on eliminating lattice defects in core-shell syntheses and opportunities opened for achieving superior catalytic performance. Ordered structural transition from ruthenium hcp to platinum fcc stacking sequence at the core-shell interface is achieved via a green synthesis method, and is verified by X-ray diffraction and electron microscopic techniques coupled with density functional theory calculations. The single crystalline Ru cores with well-defined Pt bilayer shells resolve the dilemma in using a dissolution-prone metal, such as ruthenium, for alleviating the deactivating effect of carbon monoxide, opening the door for commercialization of low-temperature fuel cells that can use inexpensive reformates (H 2 with CO impurity) as the fuel. One major goal in electrocatalysis studies is to produce highly active, durable catalysts, while minimizing the use of precious noble metals, especially platinum (Pt). This is the key requirement for the large-scale commercialization of proton exchange membrane (PEM) fuel cells [1] , [2] . An effective approach is to fabricate core-shell nanoparticles (NPs) that have active, corrosion-resistant Pt atoms on the surface, with tunable reactivity through their interactions with other metal cores to assure optimal catalytic performances. At the cathode, Pt monolayer (ML) catalysts with Pd or Pd 9 Au alloy cores exhibited enhanced activity and durability for the oxygen reduction reaction compared with Pt NPs [3] . Furthermore, both experimental and theoretical studies verified that lattice contraction [4] , [5] , [6] , [7] , high-coordination (111) facets [8] , [9] , [10] and smooth surface morphology [11] are beneficial structural factors in enhancing oxygen reduction reaction activity and the catalysts’ durability. For the hydrogen oxidation reaction (HOR) at the anode, a negligible overpotential loss was achieved with pure hydrogen using 50 μg cm −2 Pt NPs [12] , [13] . However, the challenge remains in employing inexpensive reformate hydrogen, wherein the p.p.m.-level of carbon monoxide (CO) impurities can severely deactivate the Pt catalysts [14] , [15] , [16] . In addition, although the anode operates at relatively low potentials, its nanocatalysts must be dissolution resistant because of the high potentials experienced during startups and shutdowns [17] , [18] . For developing CO-tolerant HOR catalysts, ruthenium (Ru) was used to support spontaneously deposited sub-ML Pt [19] , [20] . With about a one- to two-ML-thick Ru(core)–Pt(shell) (denoted as Ru@Pt) NPs, theoretical calculations and temperature-programmed measurements showed preferential CO oxidation in hydrogen feeds on Ru@Pt NPs compared with that of Ru–Pt nano-alloys [21] and of Pt shells with other metal core [22] . Besides being a promoter of CO tolerance of Pt surface, Ru is less expensive than Pt, but it is prone to dissolution under oxidative conditions. Thus, our elaborating well-defined Ru@Pt NPs with complete, uniform Pt shells opens an opportunity to achieve the CO tolerance and corrosion resistance needed for commercializing reformate-fed PEM fuel cells. The central issue here is to obtain uniform Pt shells with thicknesses tunable in the one to three ML range using economically viable synthesis methods. Surface science studies of Pt thin films on Ru(0001) surfaces revealed a significant increase of CO binding energy on the Pt surface, from 0.99 eV on an ML to 1.21 eV on a bilayer, and about 1.30–1.35 eV for ≥3 MLs [23] , along with a remarkable variation of oxygen adsorption behaviour on one- to three-ML-thick Pt films [24] . These profound thickness-dependent effects suggest the need and the opportunity for advancing the HOR catalysts’ CO tolerance and corrosion resistance via precisely controlling the thickness of well-defined Pt shells. However, it was questioned whether a sharp Ru–Pt core-shell interface is possible at the atomic level, because Ru cores were considered disordered in previously synthesized Ru@Pt NPs based upon the commonly observed weak Ru intensities in their X-ray diffraction (XRD) profiles [21] , [25] . Here we develop an economically viable method for reliably producing well-ordered Ru@Pt NPs. With in-depth characterizations and analyses of the hcp to fcc structural phase transition at the Ru–Pt core-shell interface, we find that defect-induced partial alloying is the cause of Ru disordering, and so succeed in fabricating single crystalline Ru@Pt NPs with well-defined, energetically favourable hcp to fcc structural transition at the core-shell interface. The significance of this achievement is demonstrated by the superior durability and excellent CO tolerance of the bilayer-thick Ru@Pt nanocatalysts for the HOR in PEM fuel cells at ultra-low catalyst loadings (25 μg cm −2 Pt, 10 μg cm −2 Ru). The results hold great promise for using low CO content reformates without much penalty in performance with the cost of catalyst comparable with that of the 50–100 μg cm −2 Pt currently used for pure hydrogen fuel cells. This change would engender considerable savings in operating hydrogen fuel cells, because the 2,015 price target for hydrogen produced by reforming natural gas is $2 per kg H 2 , viz., ~40% cheaper than pure hydrogen generated by water electrolysis at $3.5 per kg H 2 (ref. 26 ). Synthesis of well-defined core-shell NPs We used the solvent ethanol as the reductant, without any other organic agents or metal templates, to fabricate Ru NPs and to coat them with Pt atomic layers. The processes of metal deposition were manipulated via fine-tuning the reducing power of ethanol. In reacting with metal ions, ethanol itself is oxidized: first, to acetaldehyde by removing two H atoms and then to acetic acid by adding one O atom, giving up two electrons at each step ( Fig. 1a ). 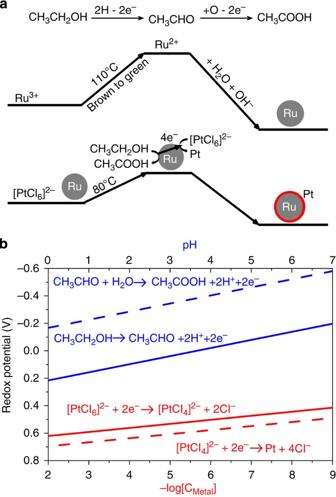Figure 1: Core-shell nanosyntheses with solvent ethanol as the reductant. (a) Schematic illustration of the synthesis routes for Ru NPs and for coating them with Pt, as well as the two steps of ethanol oxidation. (b) Standard redox potentials at 23 °C as a function of pH and metal precursors’ concentrations, in which the slopes=−2.303 RT/nF, with 0.059 V per pH and 0.0295 V per decade concentration for Pt complexes, because one electron transfer per H+and two for Pt ions. The values at pH 7 are −0.197 V for ethanol/acetaldehyde and −0.58 V for acetaldehyde/acetate54. The values for 1 M PtCl62−/PtCl42−and PtCl42−/Pt are 0.68 and 0.755 V, respectively55. Figure 1b shows the pH-dependent redox potentials for these two reactions. The more negative the value is, the higher is the reducing power. Therefore, the intermediate, acetaldehyde, is a less stable, stronger reductant than ethanol. This fact leads to a considerable activation barrier for the first step of ethanol oxidation; thus, noble-metal precursors that have more positive reduction potentials than ethanol can be dissolved and uniformly mixed with the reductant without being reduced at ambient temperature. Adding water or an alkaline solution that affords a source of oxygen enables the second step, whereas increasing the pH facilitates both reactions. Thus, we can use temperature, H 2 O and pH as the tuning knobs to control the synthesis process. Compared with other synthesis methods, we found that simplicity leads to high reproducibility and scalability. The results, virtually 100% metal yield with ethanol as the sole solvent and reductant, clearly show the commercial value of the method. Figure 1: Core-shell nanosyntheses with solvent ethanol as the reductant. ( a ) Schematic illustration of the synthesis routes for Ru NPs and for coating them with Pt, as well as the two steps of ethanol oxidation. ( b ) Standard redox potentials at 23 °C as a function of pH and metal precursors’ concentrations, in which the slopes=−2.303 RT/nF, with 0.059 V per pH and 0.0295 V per decade concentration for Pt complexes, because one electron transfer per H + and two for Pt ions. The values at pH 7 are −0.197 V for ethanol/acetaldehyde and −0.58 V for acetaldehyde/acetate [54] . The values for 1 M PtCl 6 2− /PtCl 4 2− and PtCl 4 2− /Pt are 0.68 and 0.755 V, respectively [55] . Full size image In synthesizing Ru NPs, we first refluxed ethanol solutions containing RuCl 3 metal precursors (pH~1) at 110 °C for 1 h. The colour of the solution changed from brown (Ru 3+ ) to green (Ru 2+ ) without the formation of Ru metal particles, whereas ethanol oxidation was limited to the first step because of the lack of an oxygen source. A fast nucleation process was then initiated by adding an aqueous alkaline solution to enable the second-step oxidation of ethanol, resulting in the formation of Ru NPs. The molar amount of OH − is three times that of Ru 3+ ions, which equals to the amount of protons generated by the reaction at one proton per electron transfer. This condition eliminates the formation of any Ru hydroxide or oxide. The carbon-supported Ru NPs were synthesized by adding either carbon powder (C) or carbon nanotubes (CNTs) before adding an aqueous alkaline solution. This synthetic route resulted in a uniform dispersion and strong bonding between the Ru and carbon supports. For fabricating atomically ordered core-shell NPs, we further annealed the supported Ru NPs in hydrogen at 350–500 °C to minimize lattice defects and the number of particles with diameters less than 2 nm. Typical low-magnification images are shown in Supplementary Fig. S1 . To coat atomic layers of Pt on Ru NPs, we used an ethanol solution containing H 2 PtCl 6 that is stable at room temperature. In the absence of Ru NPs, Pt deposition on carbon did not occur below 100 °C. For the Ru@Pt NPs fabricated with Pt coating temperature ≤80 °C, we verified the absence of Pt-only particles using the Ru:Pt ratio of individual particles determined by energy-dispersive X-ray spectroscopy. The optimal coating for seed-mediated Pt deposition on Ru occurred at 80 °C. This temperature is sufficiently low to avoid Pt nucleation, yet high enough to dominate Pt reduction via the oxidation of ethanol rather than of Ru. In an aqueous solution without reducing agents, Pt ions can be deposited through galvanic replacement of Ru, a metal that is less noble than Pt [27] ; this is an undesirable reaction, as it could cause loss of Ru or result in Ru–Pt mixed shells [28] . At 80 °C, the [PtCl 6 ] 2− ions usually had become colourless in 2–3 h; we note that to ensure the completion of Pt deposition, an aqueous alkaline solution may be added up to twice the molar amount of Pt precursors. After filtration, we confirmed, by energy-dispersive X-ray fluorescence measurements, that there were negligible amount of Ru and Pt ions in the solutions. By adjusting the amount of the Pt precursor and average size of the Ru particles, we synthesized and structurally characterized the Ru@Pt samples with Pt shell thicknesses ranging from one to three atomic layers. Structural characterization and analyses Ru and Pt have different crystalline structures, thus allowing us to distinguish whether the Ru–Pt core-shell boundary is well defined. Ru(hcp) and Pt(fcc), both consist of closely packed planes of atoms, differing in their stacking sequence: The hcp layers cycle between two shifted positions, expressed as ABAB, whereas the fcc layers cycle between all three equivalent shifted positions, that is, ABCABC. Their distinctive XRD features were used in previous studies to distinguish the Ru@Pt core-shell NPs, synthesized by using a sequential polyol process at 200 °C, from the Ru–Pt alloy NPs [21] , [25] . We obtained a similar XRD profile for the Ru@Pt sample prepared with the as-synthesized Ru cores ( Fig. 2a , purple curve). It differs from that for pure Pt NPs by the notable intensity between the fcc Pt (111) and (200) peaks, originating from the hcp-Ru (002) and (101) diffractions. Because of the relative weakness of the hcp diffractions, the Ru cores were considered to be highly disordered [25] . 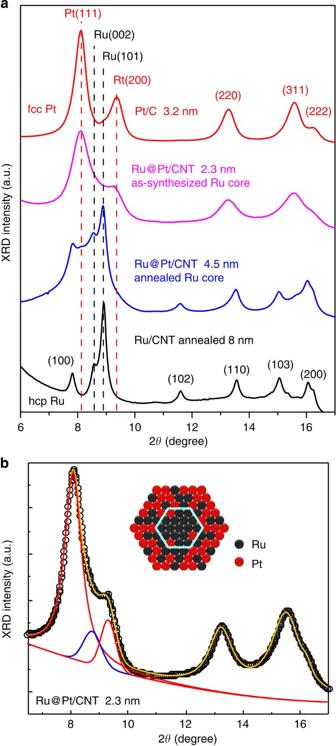Figure 2: XRD of mono- and bimetallic NPs. (a) XRD intensity profiles measured with synchrotron beamλ=0.3196 Å showing, respectively, the fcc-dominant and hcp-dominant structures for the Ru@Pt1.0NPs made with as-synthesized Ru cores (purple) and annealed ones (blue) in comparison with that of Ru (black) and Pt (red) NPs. The average sizes of the NPs were obtained by TEM measurements (Supplementary Fig. S1), and the average Pt shell thicknesses were calculated from the particle size and Ru:Pt atomic ratio, assuming a well-defined core-shell structure. (b) XRD refinement (yellow line) to the fcc-dominant intensity profile (black circles) based on Pseudo–Voigt function (the combination function of Gaussian and Lorentz functions) using the Trust–Region method. The blue curve shows the shifted hcp-Ru(101) peak, and the red curves show the fcc-Pt(111) and fcc-Pt(200) peaks. Inset shows a schematic model of a partially alloyed particle that has a Ru-rich hcp core marked by the cyan line and a Pt-rich fcc shell. Figure 2: XRD of mono- and bimetallic NPs. ( a ) XRD intensity profiles measured with synchrotron beam λ =0.3196 Å showing, respectively, the fcc-dominant and hcp-dominant structures for the Ru@Pt 1.0 NPs made with as-synthesized Ru cores (purple) and annealed ones (blue) in comparison with that of Ru (black) and Pt (red) NPs. The average sizes of the NPs were obtained by TEM measurements ( Supplementary Fig. S1 ), and the average Pt shell thicknesses were calculated from the particle size and Ru:Pt atomic ratio, assuming a well-defined core-shell structure. ( b ) XRD refinement (yellow line) to the fcc-dominant intensity profile (black circles) based on Pseudo–Voigt function (the combination function of Gaussian and Lorentz functions) using the Trust–Region method. The blue curve shows the shifted hcp-Ru(101) peak, and the red curves show the fcc-Pt(111) and fcc-Pt(200) peaks. Inset shows a schematic model of a partially alloyed particle that has a Ru-rich hcp core marked by the cyan line and a Pt-rich fcc shell. Full size image We attribute the weak Ru diffraction to the formation of a Pt-rich shell on a Ru-rich core due to Ru–Pt partial alloying at the interface. Figure 2b shows the refinement of XRD, wherein the strongest (101) peak for hcp-Ru is shifted to a position corresponding to a 1.3% lattice expansion from the bulk Ru lattice spacing of 2.056–2.082 Å. As the mismatch in spacing between hexagonal layers for Pt to Ru is 5.8%, the ratio 1.3/5.8=0.22, yields an estimated Pt atomic content in a Ru–Pt alloy based on Vegard’s law [29] . This value is close to the Pt content in a Ru 5 Pt alloy (1/6=0.17). For the 1.5-nm Ru–Pt alloy NPs, the dominant lattice structures were hcp and fcc, respectively, for a Pt content ≤17% (Ru 5 Pt) and ≥50% (Ru–Pt), with twined fcc found in between, for example, 25% (Ru 3 Pt) [30] . Thus, the observed expansion in the hcp structure likely reflects the maximum lattice expansion beyond which the hcp to fcc structural transition occurs. As illustrated in Fig. 2b (inset), partially alloyed NPs with an inwardly decreasing Pt content (red dots) can account for the observed XRD feature: weak and shifted hcp-Ru diffractions from a small Ru-rich core (Pt≤22%), and intense fcc diffractions from a Pt-rich shell that is thicker than the nominal value calculated for a well-defined core-shell structure. Guided by the understanding that partial alloying occurred at the core-shell interface, we annealed the Ru NPs before coating Pt to reduce lattice defects in the Ru cores, knowing that defect-mediated diffusion has a low energy barrier, and thus promotes interlayer diffusion [31] . Remarkable improvements were observed with annealed Ru cores. We denote the carbon-supported NPs as Ru/C or Ru/CNT. With the Ru@Pt/CNT samples (1:1 atomic ratio, 4.5 nm average diameter), we obtained hcp-dominant XRD profile (the blue curve in Fig. 2a ), clearly indicating that the Ru cores were highly ordered. Higher dispersion and smaller particles were found on C than on CNT supports. For four Ru@Pt/C samples whose Pt:Ru atomic ratios were increased from 0.5 to 1.33, we show in Fig. 3 the rise in intensities at the Pt peak positions, whereas the Ru diffraction intensities were normalized to that before the Pt coating (black curves). Even with Pt:Ru≥1, the intensity at Ru(101) position is higher than that at the Pt(200) position for particles less than 4 nm in diameter, which never was the case for previously synthesized Ru@Pt [21] , [25] , [27] , [28] . These distinct features support our new belief that an atomically sharp core-shell boundary can be achieved for hcp-Ru cores with fcc Pt shells. 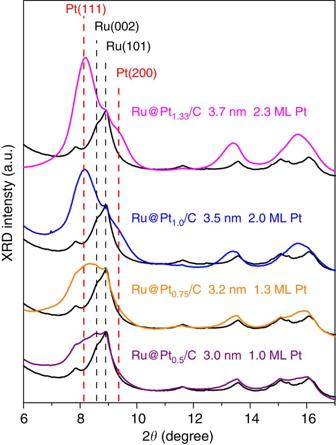Figure 3: XRD of ordered Ru@Pt NPs. Ru@Pt/C samples were made with annealed Ru cores (black curve) and the Pt:Ru ratio increased from 0.5 to 1.33. The intensities of coloured curves are normalized to the black ones at the Ru(101) position. Average particle size slightly increases with higher Pt:Ru ratio largely is due to Pt shell thickening. Figure 3: XRD of ordered Ru@Pt NPs. Ru@Pt/C samples were made with annealed Ru cores (black curve) and the Pt:Ru ratio increased from 0.5 to 1.33. The intensities of coloured curves are normalized to the black ones at the Ru(101) position. Average particle size slightly increases with higher Pt:Ru ratio largely is due to Pt shell thickening. Full size image Next, we verified the core-shell elemental distribution of individual particles at the atomic scale using various (scanning) transmission electron microscopy ((S)TEM) techniques, including a high-angle annular dark field (HAADF)–STEM and electron energy loss spectroscopy (EELS) [32] . 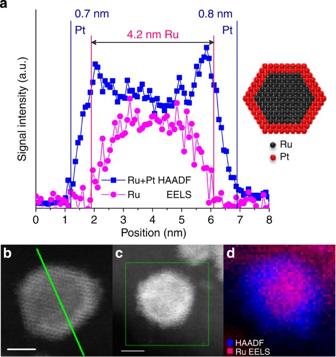Figure 4: Well-defined Ru@Pt core-shell NPs. (a) Line-scan profiles of HAADF STEM and Ru’s EELS for an ordered Ru@Pt NP. The schematic model shows a well-defined core-shell particle. (b) STEM image for the particle measured by line scan ina. Scale bar, 2 nm. (c) STEM image for the particle measured by 2D mapping ind. Scale bar, 2 nm. (d) 2D mapping of an ordered Ru@Pt NP, which is attached on carbon at the top-right corner. Figure 4a shows the intensity profiles in a line scan across a sphere-like Ru@Pt NP ( Fig. 4b ), wherein the EELS signal for Ru indicates a 4.2-nm Ru core inside a 5.7-nm NP, as measured by the HAADF. The Pt shell is about three MLs thick, as is expected for 1:1 Ru@Pt NPs with an average diameter of 5.5 nm. For another particle ( Fig. 4c ), the HAADF–EELS two-dimensional (2D) mapping ( Fig. 4d ) shows a rather uniform Pt shell around the Ru core. Figure 4: Well-defined Ru@Pt core-shell NPs. ( a ) Line-scan profiles of HAADF STEM and Ru’s EELS for an ordered Ru@Pt NP. The schematic model shows a well-defined core-shell particle. ( b ) STEM image for the particle measured by line scan in a . Scale bar, 2 nm. ( c ) STEM image for the particle measured by 2D mapping in d . Scale bar, 2 nm. ( d ) 2D mapping of an ordered Ru@Pt NP, which is attached on carbon at the top-right corner. Full size image To assist the analysis of lattice structure at the Ru–Pt core-shell interfaces, we carried out density functional theory (DFT) calculations. Focusing on the effect of the stacking sequence, we used slab models composed of four Ru layers and one or two Pt layers with a (2 × 2) hexagonal array within each layer. The atoms in the Pt layers and the top two Ru layers were relaxed. For a Pt ML, we found that the energy is slightly lower for the Ru(ABAB)-Pt(C) sequence (−33 meV) than for that of Ru(ABAB)–Pt(A) ( Supplementary Table S1 and Supplementary Fig. S2 ). Adding a second Pt layer with two choices for each type of ML creates four possible stacking sequences. The DFT calculations revealed that two of them have lower energies than the all-hcp-Ru(ABAB)–Pt(AB) sequence. One is the Ru(ABAB)-Pt(AC) sequence (−160 meV); the other is the Ru(ABAB)–Pt(CA) sequence (−134 meV). The side views of these structure models are depicted in Fig. 5a . 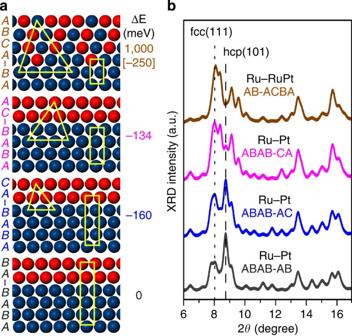Figure 5: Optimized stacking sequences with simulated XRD. (a) Favourable stacking sequences for two layers of Pt (red) on four layers Ru (blue) slab models. The differences in energy, ΔE, are given relative to the bilayer model with the all-hcp sequence, Ru(ABAB)–Pt(AB), shown at the bottom. The additional ΔEvalue in square bracket for the partially alloyed model at the top is with respect to the partially alloyed model with all-hcp sequence, that is, Ru(AB)–RuPt(ABAB). The number of layers involved in fcc–ABC and hcp–AB sequences are highlighted, respectively, by the yellow triangles and rectangles. (b) Simulated XRD using the structural models ina, illustrating the effect of the stacking sequence on the relative intensities at the fcc-(111) and hcp-(101) positions. Atomic factors and the effects of lattice stain and particle size are not included. Figure 5: Optimized stacking sequences with simulated XRD. ( a ) Favourable stacking sequences for two layers of Pt (red) on four layers Ru (blue) slab models. The differences in energy, Δ E , are given relative to the bilayer model with the all-hcp sequence, Ru(ABAB)–Pt(AB), shown at the bottom. The additional Δ E value in square bracket for the partially alloyed model at the top is with respect to the partially alloyed model with all-hcp sequence, that is, Ru(AB)–RuPt(ABAB). The number of layers involved in fcc–ABC and hcp–AB sequences are highlighted, respectively, by the yellow triangles and rectangles. ( b ) Simulated XRD using the structural models in a , illustrating the effect of the stacking sequence on the relative intensities at the fcc-(111) and hcp-(101) positions. Atomic factors and the effects of lattice stain and particle size are not included. Full size image At the top, we show one partially alloyed model in which the Pt atoms were distributed among the top four layers with their Pt concentration varying from 3/4, 2/4 and 2/4 to 1/4 (three-dimensional model in Supplementary Fig. S3 ). The energy for the Ru(AB)–RuPt(ACBA) partial-alloy model is much higher than those of the Pt bilayer models (for example, 1,000 meV relative to the Ru(ABAB)–Pt(AB) model), indicating that the Pt atoms preferentially stay on top of the Ru surfaces, consistent with the predication based on calculated surface segregation energies [33] . Driven by entropy and with the presence of steps on real surfaces, disordered surface alloys were observed when the Ru(0001) crystals with a 0.5 to 1 Pt ML were annealed at temperatures between 800 and 1,350 K [34] . For NPs, interlayer diffusion can happen at even lower temperatures, especially on defect-rich ones. When alloying occurs, the Ru(AB)–RuPt(ACBA) stacking sequence is more favourable by −250 meV than that of the Ru(AB)–RuPt(ABAB). To characterize the structural models in Fig. 5a , we drew the yellow rectangles to show how many layers have atoms at the same positions as the ones in the second layer below them. These layers are stacked in the hcp’s ABAB sequence. On the other hand, the yellow triangles mark how deep the triangular symmetry extends from the surface. The layers involved in the triangle are repeated every three layers, that is, they follow the fcc’s ABCABC stacking sequence. Figure 5b shows that the simulated XRD intensities increase at the fcc-(111) position with the number of layers in the triangles, whereas the hcp-(101) intensity is associated with the number of layers in the rectangles. These results illustrate that the ratio of the fcc-(111) to hcp-(101) intensity varies with the lattice structure at the core-shell interface. Furthermore, a partial alloy favours the fcc structure, and thus causes the XRD to be more fcc-like, consistent with experimental observation ( Figs 2 and 3 ). Complementary to XRD that provides a global monitor of the core-shell lattice structure in reciprocal space, we present below our real-space observations of the two favourable DFT-optimized hcp – fcc interfaces for the bilayer-thick Ru@Pt samples. For the particles that have the crystallographic orientation shown in Fig. 6a , the shifts in stacking sequence is denoted by the positions of the red dots with respect to the hcp sites marked by light blue circles in the ‘C’ row and the one above it. The shift can involve the top one (left part) or two (right part) layers. In other words, the first Pt layer can occupy either the C or A site with little energy difference (33 meV), a fact that is supported by an experimental observation of Pt sub-ML islands in two orientations associated with fcc and hcp stacking sequence on the Ru(0001) single crystal surface [34] . We excluded the scenario wherein a Ru layer is shifted, because the energy cost for such a shift is high, that is, 466 or 612 meV ( Supplementary Table S1 ). In addition, the spacing of the Pt layer is visibly larger than that of Ru along the surface normal direction. 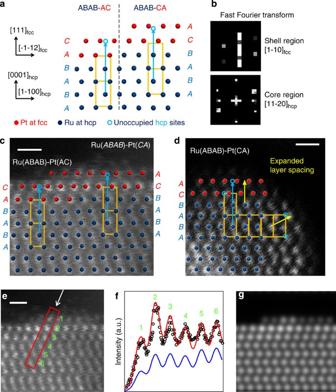Figure 6: Ordered Ru(hcp)-Pt(fcc) phase transition at core-shell interfaces. (a) Orientation of crystallographic planes for the STEM image inc, and two DFT-optimized structural models for close-packed Pt bilayer on an Ru(0001) surface. (b) Fast Fourier transform of the image inc. (c,d) HAADF STEM images and superimposed DFT-optimized structural models (red and blue dots). Scale bar, 0.5 nm. The shifts from the hcp to the fcc lattice sites at the top one or two layers are indicated by yellow rectangles, light blue circles and light blue arrows. The yellow arrows indpoint to the expanded lattice spacing along the surface normal directions. (e) The same STEM image as incfor intensity analysis. Scale bar, 0.5 nm. (f) Intensity profile along the line indicated by the arrow ine(black circles) with calculated curves using Ru@Pt core-shell (red line) and all-Ru (blue line) models. (g) Calculated STEM image based on the Ru@Pt model shown inSupplementary Fig. S4. Figure 6: Ordered Ru(hcp )-Pt( fcc) phase transition at core-shell interfaces. ( a ) Orientation of crystallographic planes for the STEM image in c , and two DFT-optimized structural models for close-packed Pt bilayer on an Ru(0001) surface. ( b ) Fast Fourier transform of the image in c . ( c , d ) HAADF STEM images and superimposed DFT-optimized structural models (red and blue dots). Scale bar, 0.5 nm. The shifts from the hcp to the fcc lattice sites at the top one or two layers are indicated by yellow rectangles, light blue circles and light blue arrows. The yellow arrows in d point to the expanded lattice spacing along the surface normal directions. ( e ) The same STEM image as in c for intensity analysis. Scale bar, 0.5 nm. ( f ) Intensity profile along the line indicated by the arrow in e (black circles) with calculated curves using Ru@Pt core-shell (red line) and all-Ru (blue line) models. ( g ) Calculated STEM image based on the Ru@Pt model shown in Supplementary Fig. S4 . Full size image To verify the presence of these features on our synthesized bilayer Ru@Pt NPs, we found the particles that exhibited the distinct fast Fourier transform patterns shown in Fig. 6b , indicating that the close-packed crystalline planes are oriented normal to the imaging plane. Figure 6c,d reveals that the atomic-resolution STEM images of such oriented particles match well with the superimposed DFT-optimized structural models. For other facets, for example, the one at the top-right corner of the image in Fig. 6d , the lattice spacing of the top two layers is visibly expanded, supporting the presence of Pt shells about two MLs thick on all facets. In addition to the changes in atomic positions, we obtained evidence for the assigned Pt layers by simulating the Z -contrast STEM image in Fig. 6e , wherein the brightness of each dot represents the intensity associated with the number of electrons per atom ( Z ) and the number of atoms in the column (that is, sample thickness). As Z Pt (78) is significantly higher than Z Ru (44), the high STEM intensities near the edge of a sphere-like particle ( Fig. 6e ) support a Pt shell. Along the line indicated in Fig. 6e , the measured intensities (black circles in Fig. 6f ) are well matched with a simulated curve (red line) using a Pt bilayer model shown in Supplementary Fig. S4 . If all the atoms were Ru, the intensity would be lower near the edge owing to decreasing thickness of a sphere-like particle (blue line). On the basis of the best match between the observed STEM image ( Fig. 6e ) and the calculated one ( Fig. 6g ), we assigned the Pt layers at the particle edge in Fig. 6c , which shows that the bilayer Pt shell shifts down at the left following the curvature of the Ru core in an energetically favourable manner. Although real-space evidence for the formation of single crystalline Ru@Pt NPs with sharp, energetically favourable interfaces is provided, a question often rises on the representativeness of such particles, because only a small portion of the NPs are at the edge of carbon support and even fewer have the appropriate orientation for detailed analyses. Therefore, correlation established between atomic-resolution STEM images for the ordered hcp – fcc phase transition and the non-diminishing Ru intensity in XRD is very helpful. The latter is a global probing technique more commonly available for characterizing synthesized samples. We show next that structural perfection is vital for catalysts’ stability and for tuning surface reactivity via the thickness of the Pt shell. Catalytic performances in PEM fuel cells Ballard Power Systems assessed the performances of highly ordered Ru@Pt catalysts with low Pt loadings for the HOR in PEM fuel cells against CO tolerance and corrosion resistance, following the testing protocols for practical fuel cell applications. Although the hydrogen produced via steam reforming and the water gas shift reaction contains about 1% of CO, advances were made in lowering the CO content to about 10 p.p.m. via the preferential oxidation reaction (CO+1/2O 2 →CO 2 in excess H 2 ) [35] , [36] , thus triggering a renewed interest in developing CO-tolerant fuel cell catalysts. The target for using a 10-p.p.m. CO hydrogen is to assure that the CO-induced loss in performance is below 10%, or with air bleeding it is reduced to <1%. Air bleeding refers to injecting a small amount of air into the stream of anode fuel to promote the oxidative removal of adsorbed CO by forming CO 2 (ref. 37 ). 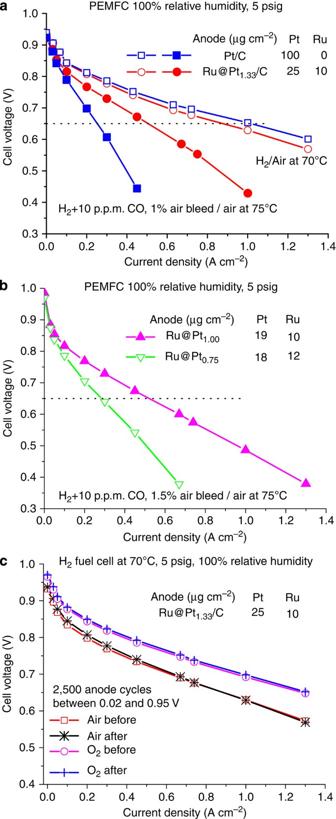Figure 7: Performance of ordered Ru@Pt/C anode nanocatalysts in PEM fuel cells. (a) Polarization curves measured with hydrogen (open symbols) and hydrogen+CO and air bleeding (solid symbols) at the anode. The cathode Pt loading was 0.4 mg cm−2and the cathode gas was air. (b) Polarization curves measured with CO-containing hydrogen for two Ru@Pt/C samples with different Pt shell thicknesses. The dotted lines inaandbare to assist comparison of the current densities at 0.65 V. (c) Catalysts’ stabilities after 2,500 anode potential cycles measured with hydrogen at the anode and air or oxygen at the cathode. The metal loadings for our core-shell catalysts were calculated using the catalysts’ weights and metals’ percentages based on the precursors used in syntheses with a 100% yield. Figure 7a shows the polarization curves obtained in hydrogen PEM fuel cells without and with CO+air bleeding. The enhanced CO tolerance on the Ru@Pt core-shell catalyst that has lower total metal loading than the Pt/C baseline is verified by the doubling of the current at 0.65 V (0.51 versus 0.25 A cm −2 ) and by the smaller decrease in current from that with pure hydrogen (−41 versus −75%). For the other two core-shell catalyst samples tested with 1.5% air bleeding ( Fig. 7b ), the current at 0.65 V is higher on Ru@Pt 1.0 /C than that on Ru@Pt 0.75 /C (0.52 versus 0.28 A cm −2 ). The average Pt shell thicknesses for the Pt:Ru atomic ratios of 0.75, 1.0 and 1.33 are, respectively, about 1.3, 2.0 and 2.3 MLs. For all the Ru@Pt samples, lattice contractions in the Pt shells ranged between −0.6 and −1.0% based on the XRD analyses ( Supplementary Table S2 ); they are expected to weaken CO adsorption [4] , [21] . Indeed, much weakened CO stripping peak was observed on the Ru@Pt 1.0 /C sample compared with that on Pt NPs ( Supplementary Fig. S5 ). However, what weakens CO adsorption also lessens the adsorption of H and O species [23] , [24] , [38] , thereby lowering the HOR activity per site and the oxidative removal of CO. Therefore, a dedicated balance is needed to assure optimal performance. We achieved that goal by using well-defined core-shell structure with a tunable shell thickness. With CO-containing H 2 , the much better performance realized on bilayer Ru@Pt NPs (solid red circles in Fig. 7a and solid purple triangles in Fig. 7b ) compared with that on the ML Ru@Pt NPs (open green triangles in Fig. 7b ) and on the Pt NPs (solid blue squares in Fig. 7a ) illustrates the importance of structural perfection for fine-tuning surface reactivity. Figure 7: Performance of ordered Ru@Pt/C anode nanocatalysts in PEM fuel cells. ( a ) Polarization curves measured with hydrogen (open symbols) and hydrogen+CO and air bleeding (solid symbols) at the anode. The cathode Pt loading was 0.4 mg cm −2 and the cathode gas was air. ( b ) Polarization curves measured with CO-containing hydrogen for two Ru@Pt/C samples with different Pt shell thicknesses. The dotted lines in a and b are to assist comparison of the current densities at 0.65 V. ( c ) Catalysts’ stabilities after 2,500 anode potential cycles measured with hydrogen at the anode and air or oxygen at the cathode. The metal loadings for our core-shell catalysts were calculated using the catalysts’ weights and metals’ percentages based on the precursors used in syntheses with a 100% yield. Full size image Corrosion resistance of the anode nanocatalysts is another important requirement for practical applications. Although the anode operates at low potentials, metal dissolution and particle agglomeration may occur owing to occasional high potentials at startup and shutdown or fuel starvation [39] . The problem is particularly detrimental for alloy Ru–Pt/C catalysts, because Ru dissolves at lower potentials than does Pt and, furthermore, Ru ions can migrate through electrolyte membranes and be redeposited at the cathode, thus depressing its activity in oxygen reduction [40] . We carried out accelerated stress tests to check the corrosion resistance of the Ru@Pt 1.33 /C sample. After 2,500 startup/shutdown cycles (~65 h) that alternated the anode’s potential between 0.02 and 0.95 V, there was little change in the polarization curves shown in Fig. 7c . This unaffected performance at the ultra-low Pt loadings signifies an excellent protection by the ordered Pt bilayer shells of the Ru cores and an enhanced stability of the Pt shells in comparison with Pt NPs. We ascribe the latter effect to Ru-induced lattice contraction and the smooth morphology obtained both by the annealed Ru cores and by coating Pt under near-equilibrium conditions to enhance the formation of energetically favourable structure. Previous studies have shown that the less reactive a surface is, the more corrosion resistant it is [7] , [8] , [11] ; low coordination sites (clusters, defects, vertices and edges) are prone to dissolution, and thus need to be minimized [8] , [11] . We demonstrate herein a case wherein lattice defects must be minimized for achieving desirable nanostructures, whereas advantages have been taken of the lattice defects and relative diffusivities of two elements to fabricate hollow nanomaterials [7] , [41] . The drastic effect of lattice defects on diffusion rate in bulk materials was noted in the 1940s [31] . Just a few per million empty sites makes the vacancy exchange the dominant mechanism for interdiffusion at the interface of two metals, because the barrier is much lower than that of direct exchange or rotation. Although interlayer mixing occurred in the Ru@Pt NPs synthesized using a sequential polyol process at 200 °C [21] , [25] , our 80 °C coating of Pt in ethanol on 450 °C-annealed Ru cores produced single crystalline Ru@Pt core-shell NPs with tunable Pt shell thicknesses as confirmed by complementary XRD and microscopy measurements. This is because the number of defects in Ru NPs is reduced by annealing at 450 °C compared with those as-synthesized at 200 °C, and the interlayer diffusion rate is further lowered by coating Pt at 80 versus 200 °C. In summary, Ru–Pt partial alloying is not inevitable for core-shell NPs with different crystal structures, and highly ordered Ru@Pt NPs with designed shell thickness can be reliably produced by a fine-tuned ethanol-based method of synthesis. This new level of atomic control in synthesis allowed us to use bilayer Ru@Pt NPs for enhancing both CO tolerance and corrosion resistance. The significantly enhanced CO tolerance and the superior stability demonstrated in accelerated stress tests at ultra-low catalyst loadings show the promise of using a well-ordered core-shell structure to resolve the dilemma in using dissolution-prone metals for alleviating the CO-poisoning effect. We note that the current at 0.65 V for the Ru@Pt/C sample with Pt loading of 25 μg cm −2 was reduced by less than half with CO-containing hydrogen than with pure hydrogen. Thus, the targeted <1% performance loss is likely achievable with total metal loading <100 μg cm −2 , which is comparable to that currently used in the hydrogen fuel cell anode. In addition to a direct saving on operational cost with less-expensive hydrogen from reforming natural gas, enabling reformates as the fuel will ease the building up of hydrogen infrastructure for commercializing PEM fuel cells. We expect that the significant advance in catalytic performance made via eliminating defects in this case will inspire further efforts in nanosyntheses to fully realize the potentials suggested by studying ideal models on single crystal surfaces for a wide range of applications. Synthesis of unsupported metal NPs In a typical synthesis of unsupported Ru NPs, a 50-ml ethanol (200 proof) solution containing 150 μmol RuCl 3 was refluxed at 110 °C for 1 h, while rigorously stirring it, during which the solution’s colour turned from brown to greenish, reflecting the partial reduction of Ru 3+ to Ru 2+ . Thereafter, we gradually added 4.5 ml 0.1 M aqueous NaOH solution (450 μmol=3 times of 150 μmol of RuCl 3 ), enabling a further reduction to metallic Ru NPs. After 2 h, we ensured the complete reduction of Ru ions by raising the pH to neutral with a little extra alkaline solution (<200 μmol). The mixture was cooled down to room temperature, filtered, rinsed and dried. Synthesis of carbon-supported metal NPs In a typical synthesis of carbon-supported Ru NPs, 100 ml ethanol solution containing 400 μmol RuCl 3 was refluxed at 110 °C with rigorous stirring for 1 h in a three-necked flask; meanwhile, 200 mg carbon powder (Ketjenblack EC-600JD) or CNTs (OH functionalized, 15 nm in diameter) were disbursed in 60 ml ethanol by sonication for 20 min. The slurry was transferred into the reaction flask with additional 10 ml ethanol to assure a complete transfer. After the temperature stabilized at 110 °C, 12 ml of a 0.2 M aqueous alkaline solution of 1,200 (3 × 400) μmol NaOH was injected, while stirring vigorously. Two hours later, the colour of the solution was checked. If it was not completely colourless, additional 0.5 × 400=200 μmol NaOH was added. The heater was turned off, allowing the mixture to cool slowly in the oil bath to room temperature before filtering it. Coating shell metal onto core NPs In a typical synthesis of Ru@Pt core-shell NPs, an as-synthesized Ru/C (400 μmol Ru) sample was annealed in H 2 at 450 °C for 1 h, dispersed in 100 ml ethanol, and refluxed at 110 °C for 1 h. After cooling to room temperature, 8 ml of 50 mM H 2 PtCl 6 (400 μmol) ethanolic solution was added, while vigorously stirring or sonicating to ensure a uniform dispersion. The mixture was heated to 80 °C and maintained there for 2 h. The solution usually became colourless; if not, up to 2 × 400 μmol NaOH was added to completely reduce Pt. The mixture was cooled to room temperature, filtered and rinsed with copious amount of water to eliminate the Cl − ions. The synthesized sample had a 1:1 Ru:Pt atomic ratio, along with 25 wt% Pt and 37 wt% Pt+Ru on carbon supports. Structural characterization STEM measurements were performed using the Hitachi HD2700C operated at 200 kV, equipped with a cold-field emission electron source and a probe aberration corrector. In a vibration-isolated and temperature-stabilized room, the spatial resolution for imaging is about 1.0 Å. The probe current was in the 50–100 pA range. The sample for STEM was prepared by drop casting the ethanolic suspension of carbon-supported NPs on a carbon-coated copper grid (Lacey carbon support film, 300 mesh, Ted Pella Inc.). We took the Z n -contrast ( Z is the atomic number and n is ~1.7) [42] STEM images using a HAADF detector. Elemental line scans and 2D mappings were made with a high-resolution EELS detector (Gatan Enfina-ER). We employed a convergence semi-angle of 28 mrad. With an energy dispersion of 0.3 eV per channel and a collection semi-angle of 20 mrad, the energy resolution was around 0.45 eV. The exposure time for each spot was about 0.07 s with a step size of 0.9 Å for EELS line scans and was 0.05 s for 2D mapping. We extracted the Ru EELS signal from the EELS spectrum using a power-law background model and an integration window at the Ru M 4,5 edge [43] , [44] . The STEM image simulations were carried out with our own computer codes running on GPU based on the multislice method with a frozen phonon approximation. The calculated STEM images were convoluted with a 0.15-nm full-width half maximum Gaussian spread function for comparison with experiments. TEM images were taken with a JEOL 3000F TEM operating at 300 kV, equipped with Gatan image filter system. XRD experiments were carried out on beamline X7B ( λ =0.3196 Å) of the National Synchrotron Light Source at Brookhaven National Laboratory. Two-dimensional powder patterns were collected with a PerkinElmer image plate detector, and the diffraction rings were integrated using the FIT2D code. Lanthanum hexaboride (LaB6) was used as the instrumental reference. We refined the fits to the XRD peaks based on the Pseudo–Voigt function (the combination function of Gaussian and Lorentz functions) using Trust–Region method. Computational methods The calculations were performed by using periodic DFT as implemented in the Vienna ab-initio simulation package [45] , [46] . Ion-core electron interactions were described using the projected augmented wave method [47] , [48] , and the Perdew–Wang functional (GGA-PW91) within the generalized gradient approximation [49] , [50] was used to describe exchange-correlation effects. The cutoff energy of plane-wave basis set was 400 eV. The five- or six-layer slab models have four atoms in a (2 × 2) hexagonal array within each layer, and a vacuum of 12 Å between the slabs. The 9 × 9 × 1 k -points using the Monkhorst–Pack scheme [51] and first-order Methfessel—Paxton smearing [52] of 0.2 eV was employed in the integration to speed up the convergence. The conjugate gradient algorithm was used for optimization, allowing the convergence of 10 −4 eV in total energy and 10 −3 eV Å −1 in Hellmann–Feynman force on each atom. All atoms were allowed to relax, except those of the bottom two layers that were fixed at the hcp-Ru bulk position with the optimized lattice constant of a = b =2.731 and c =4.307 Å. Simulated XRD spectra were obtained using Reflex module embedded in Materials Studio 5.5 by Accelrys ( http://accelrys.com/products/materials-studio/ ) with X-ray source being a synchrotron beam ( λ =0.3196 Å) as in the experimental measurements, step size of 0.01° and Pseudo–Voigt broadening of 0.1°. Fuel cell tests Fuel cell accelerated stress tests for the anodes were carried out on membrane electrode assemblies with an active electrode area of 45 cm 2 . The cathode catalyst was Pt/C (Pt loading: 0.4 mg cm −2 ), the membrane was Nafion211 and the gas diffusion layers were obtained from Ballard Material Products. During the accelerated stress test, the fuel cell was alternated between operating (1 A cm −2 ) and shutdown modes, with the anode potential cycled between ~0.02 V and ~0.95 V, and the cathode potential cycled between ~0.55 V and ~0.93 V (ref. 53 ). In-situ cyclic voltammetry measurements for CO stripping were performed using CorrWare software with a PAR Model 263A potentiostat connected to a 20-A Kepco power booster, by flowing hydrogen on the cathode (acting as a pseudo hydrogen reference electrode) and nitrogen on the anode. How to cite this article: Hsieh, Y.-C. et al. Ordered bilayer ruthenium–platinum core-shell nanoparticles as carbon monoxide-tolerant fuel cell catalysts. Nat. Commun. 4:2466 doi: 10.1038/ncomms3466 (2013).